2q36.3 is associated with prognosis for oestrogen receptor-negative breast cancer patients treated with chemotherapy Large population-based registry studies have shown that breast cancer prognosis is inherited. Here we analyse single-nucleotide polymorphisms (SNPs) of genes implicated in human immunology and inflammation as candidates for prognostic markers of breast cancer survival involving 1,804 oestrogen receptor (ER)-negative patients treated with chemotherapy (279 events) from 14 European studies in a prior large-scale genotyping experiment, which is part of the Collaborative Oncological Gene-environment Study (COGS) initiative. We carry out replication using Asian COGS samples ( n =522, 53 events) and the Prospective Study of Outcomes in Sporadic versus Hereditary breast cancer (POSH) study ( n =315, 108 events). Rs4458204_A near CCL20 (2q36.3) is found to be associated with breast cancer-specific death at a genome-wide significant level ( n =2,641, 440 events, combined allelic hazard ratio (HR)=1.81 (1.49–2.19); P for trend=1.90 × 10 −9 ). Such survival-associated variants can represent ideal targets for tailored therapeutics, and may also enhance our current prognostic prediction capabilities. We have previously shown, through large population-based registry studies, that survival from breast cancer is correlated among relatives, consistent with an inherited cancer prognosis [1] , [2] , [3] , [4] . A potential explanation for the heritability of survival would be that family members are predisposed to developing a breast cancer tumour of predefined aetiology and predetermined tumour characteristics. This is plausible given the observation that carriers of high- and moderate-risk germline mutations in genes such as BRCA1 , BRCA2 , CHEK2 and PALB2 , are predisposed to specific subtypes of breast cancer [5] , [6] , [7] , [8] , and that many common variants identified through genome-wide association studies (GWAS) tend to be associated with specific subtypes, with some variants more strongly associated with oestrogen receptor (ER)-negative or triple-negative breast cancer [9] , [10] , [11] , while others more strongly associated with ER-positive breast cancer [12] , [13] , [14] . It is also possible that the inherited predeterminants of survival lie not in the biology of the tumour but rather the milieu in which the tumour arises. The tumour microenvironment is composed of tumour cells, fibroblasts, endothelial cells and infiltrating immune cells, which may inhibit or promote tumour growth and progression. There is empirical support for the concept that a host immune response might enhance the effects of conventional chemotherapy, conceivably having an influence on breast cancer outcome. For example, the presence of tumour-associated lymphocytes in a breast tumour has been suggested to be an independent predictor of neoadjuvant chemotherapy response [15] . Other studies have shown the host immune system to be involved in the elimination of tumour cells to control cancer growth [16] , [17] . In this candidate pathway study, we investigate the pre-specified hypothesis that the germline common variants of genes involved in immune response and inflammation can predict the response to breast cancer survival for ER-negative, chemotherapy-treated patients. We identify a single-nucleotide polymorphism (SNP) near the CCL20 gene (2q36.3), which is associated with a difference in the clinical outcome of ER-negative breast cancer treated with chemotherapy independent of known tumour prognostic features. Individual patient-level genetic and phenotypic data were extracted from European studies in a prior large-scale genotyping experiment conducted in the Breast Cancer Association Consortium (BCAC), part of the Collaborative Oncological Gene-environment Study (COGS) initiative [18] . For this study, we selected women of European descent inferred from genetic ancestry with invasive breast cancer, who have had no previous diagnosis of the disease. Subjects missing follow-up information on vital status, time to vital status, date of study entry and cause of death data were excluded. The selection of only ER-negative patients in this study was strongly motivated by prior insight. A Swedish study of the breast cancer prognosis of 834 sister pairs in which both were affected showed that younger sisters with poor older sister survival had worse survival than younger sisters with good older sister survival (number of breast cancer deaths within 5 years from diagnosis in younger sisters, n event =65, P =0.02 in a multivariate proportional hazard (Cox) analysis) [3] . When stratified by ER subtypes, the increased risk of death from ER-negative breast cancer for younger sisters with poor older sister survival compared with younger sisters with good older sister survival was found to be almost sevenfold ( n =139 sister pairs, n event =28, hazard ratio (HR)=6.69 (1.36–32.91), P =0.02) in contrast to sister pairs with the ER-positive disease ( n =584 sister pairs, n event =28, HR=1.54 (0.48–4.98), P =0.50) (unpublished data). In addition, in a recent Breast International Group phase III trial, increasing lymphocytic infiltration was found to be associated with excellent prognosis only for patients with node-positive, ER-negative/HER2-negative disease [19] . 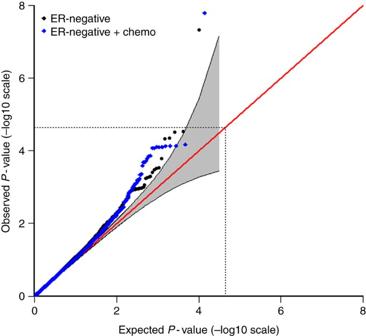Figure 1: Quantile–quantile (QQ) plots of the observedP-values for association in the discovery stage. QQ plot of the observed −log10P-values (yaxis) versus the ‘expected’ −log10 rankP-values (xaxis) for trend tests of association of 7,020 human immunology and inflammation SNPs, with the risk of dying from breast cancer for all ER-negative breast cancer patients (black/below) and ER-negative patients treated with adjuvant chemotherapy (blue/above) (genomic inflation factor,λ=1.16 and 1.14, respectively) in the discovery phase. The grey region indicates bootstrapped 95% confidence intervals. The diagonal red line indicates expected results under null hypothesis. The dotted lines indicate Bonferroni threshold for multiple-testing correction (2,184 independent tests withr2<0.2). Twenty studies with ER-negative cases and at least one event (breast cancer-specific death) were eligible for the combined analysis ( Supplementary Table 1 ). As we were primarily interested in response to chemotherapy, patients missing information on chemotherapy were not considered in our analyses. 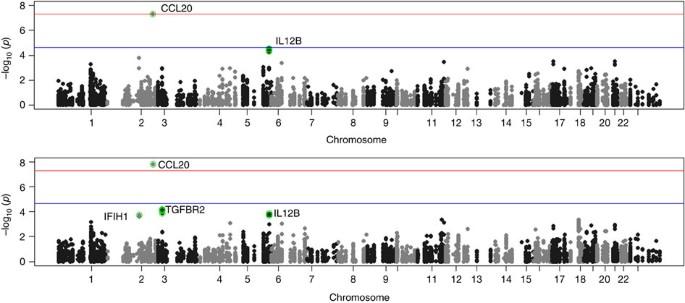Figure 2: Manhattan plot for association in the discovery stage. Manhattan plot showing directly genotyped SNPs plotted according to chromosomal location (xaxis), with −log10P-values (yaxis) derived from trend tests of association of 7,020 human immunology and inflammation SNPs with the risk of dying from breast cancer for all ER-negative patients (above) and ER-negative patients treated with chemotherapy (below) in the discovery phase. Blue and red lines indicate the Bonferroni threshold for multiple-testing correction for 2,184 (r2<0.2) and genome-wide significance level (5 × 10−8), respectively. SNPs with FDRs of <10% are additionally encircled and denoted in green. Chromosomal positions are based on NCBI build 36. The 14 studies ( n =1,804) included in the combined analysis for the chemotherapy-treated subgroup are summarized in Supplementary Table 2 . A total of 279 breast cancer-specific deaths were recorded in a 15-year follow-up. 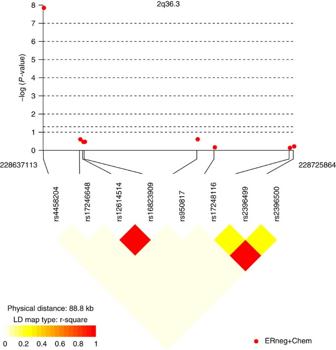Figure 3: Linkage disequilibrium plot of SNPs within a 100-kb window flanking rs4458204 in the discovery phase. The closest SNP flanking the left of rs4458204 is >9.5 Mb away. Chromosomal positions are based on NCBI build 36.P-values are derived from trend tests of association. Plotted using ‘snp.plotter’ package in R. For the replication phase, four iCOGS Asian studies with ER-negative breast cancer cases treated with chemotherapy and at least one death due to breast cancer in a 15-year follow-up were analysed ( n =522, 53 events, Supplementary Table 3 ). Early-onset breast cancer patients from the independent Prospective Study of Outcomes in Sporadic versus Hereditary breast cancer (POSH) study [20] , [21] were used as a second replication data set. In particular, we performed our replication using ER-negative breast cancer patients treated with chemotherapy in the POSH study’s Stage 1 discovery data set samples ( n =315, 108 events) selected to facilitate studies on breast cancer prognosis [22] . The breast cancer-specific death rate is thus particularly high and there were few cases that drop out due to lack of phenotype information. All women in participating studies had provided written consent for the research and approval for each study was obtained from their local ethical review board ( Supplementary Tables 1 and 3 ). Collection of blood samples and clinical data from subjects was performed in accordance with local guidelines and regulations. Genotyping was conducted using a custom Illumina iSelect genotyping array (iCOGS), comprising 211,115 SNPs. Details of quality control of the iCOGS data are described in detail elsewhere [18] . Briefly, individuals were excluded for any of the following reasons: genotypically not female XX (XY, XXY or XO), overall call rate <95%, low or high heterozygosity ( P <1 × 10 −6 , determined separately for individuals of European and East Asian ancestry), genotypes discordant with those determined in previous genotyping such that the individual appeared to be different, genotypes for the duplicate sample that seemed to be from a different individual and cryptic duplicates. SNPs with call rates of <95%, SNPs that deviated from Hardy–Weinberg equilibrium in controls at P <1 × 10 −7 and SNPs for which the genotypes were discrepant in >2% of duplicate samples across all COGS consortia were excluded. The final analyses in the parent COGS study were based on data from 199,961 SNPs. Key genes related to human immunology and inflammation were identified from two comprehensive and highly curated gene panels (nCounter GX Human Immunology Kit and nCounter GX Human Inflammation Kit, NanoString Technologies, Seattle, WA, USA), which are commercially available ( Supplementary Data 1 ). We identified all SNPs on the iCOGS within a 50-kb window of any gene on the panel. Out of 8,237 unique SNPs extracted from COGS, we further removed SNPs with low minor allele frequency (<0.05) and low call rate (<0.95). After quality-control exclusions, we analysed 7,020 non-overlapping SNPs in 557 unique gene regions (from 597 genes on the original nCounter panels). In the POSH study, rs4458204 was genotyped on the Illumina 660 W-Quad SNP array. Details can be found in the parent POSH article [22] . Briefly, genotyping for the samples was conducted in two separate batches in two locations (Mayo Clinic and the Genome Institute of Singapore). To ensure harmonization of the genotype calling, the intensity data were combined and used to generate genotypes based on the algorithm available in the genotyping module of Illumina’s Genome Studio software. Breast cancer survival, right-truncated at 15 years after diagnosis, was modelled by using multivariate Cox proportional hazard analyses, treating each SNP as an ordinal variable (that is, 0, 1 and 2 copies of minor allele). Analyses were partially adjusted for age at diagnosis (years), study and seven principal components (as recommended by COGS) as covariates. As comparisons of survival are often confounded by differences in the patients, their tumours or the treatments, we further included covariates on tumour characteristics and treatment in a fully adjusted model,which is presented as the main analysis in this study. The fully adjusted model was additionally adjusted for tumour size (≤2, >2 and ≤5, or >5 cm), presence of distant metastasis (M from the Tumour, Nodes and Metastasis (TNM) staging system), lymph node status (negative/positive), histopathological grade (well, moderately or poorly differentiated), surgery (no surgery, breast-saving or mastectomy with or without axillary), hormone therapy (Yes/No) and radiotherapy (no radiation, breast only, breast and lymph nodes or lymph nodes only). Missing values were coded separately as missing. Separate baseline hazard functions were fitted for each study. Between-study heterogeneity was evaluated by using the Q statistic and the I 2 metric [23] . Estimated HRs and confidence limits are presented for heterozygotes and minor allele homozygotes, relative to the major allele homozygotes. Delayed entry (left truncation) was allowed for all models to adjust for the timing of blood draw. The proportional hazards assumption for each SNP was assessed using Schoenfeld’s test statistics [24] . The Kaplan–Meier estimator for delayed-entry data was computed using the survfit function from the survival package in R. The Nagelkerke pseudo R -squared statistic was used to assess variance explained [25] . To adjust for multiple testing without overly penalizing the tests, we determined the number of ‘independent’ SNPs. SNPs were thinned using the ‘—indep-pairwise’ option in PLINK [26] such that all SNPs within a window size of 50 SNPs (step size of 10) were required to have r 2 <0.2. This procedure resulted in a set of 2,184 independent SNPs pruned by linkage disequilibrium. The Bonferroni-adjusted threshold for 2,184 independent tests is 2.29 × 10 −5 . In addition to standard Bonferroni adjustment, a 10% false discovery rate (FDR) threshold was applied to try to identify more candidate SNPs associated with breast cancer outcome. An FDR-adjusted P -value of 0.10 implies that 10% of significant tests will result in false positives. The results for tests of association between 7,020 human immunology and inflammation SNPs and risk of death from ER-negative breast cancer are summarized in Supplementary Data 2 and 3 . The deviation of the smaller observed P -values from those expected ( λ =1.16) is consistent with multiple weak associations between these SNPs and survival for ER-negative breast cancer patients ( Fig. 1 ). In particular, for a single SNP rs4458204_A located on chromosome 2:228637113 (minor allele frequency=0.12), the χ 2 (1df) association test statistic was much higher than for the other SNPs and was close to surpassing the threshold for experiment-wide significance after Bonferroni adjustment ( P <2.29 × 10 −5 ) in the partially adjusted analysis stratified by study and adjusted for only population stratification and age ( n =2,218, 332 events, per-allele HR=1.54 (1.26–1.90), P for trend=3.62 × 10 −5 , Supplementary Data 3 ). However, after further adjusting for appropriate patient tumour and treatment characteristics, the SNP association surpassed the threshold for genome-wide significance ( P <5 × 10 −8 ) (per-allele HR=1.83 (1.47–2.27), P for trend=4.68 × 10 −8 , Table 1 and Fig. 2 ), a conservative threshold which is likely to be overly stringent [27] . The lack of an association signal tower could be because the iCOGS was designed to have minimum linkage disequilibrium across SNPs. No SNP within a 100-kb window is correlated to rs4458204 with r2>0.2 ( Fig. 3 ). The association was stronger for a subset of ER-negative patients who had been treated with chemotherapy ( n =1,804, 279 events, per-allele HR=1.96 (1.55–2.47), P for trend=1.60 × 10 −8 ). We found no evidence of heterogeneity in the per-allele HR across 14 studies ( I 2 =0%, P for heterogeneity=0.84; forest plot in Fig. 4 ). Univariate Kaplan–Meier survival curves of breast cancer-specific survival for ER-negative patients treated with chemotherapy by rs4458204 genotypes are presented in Fig. 5 (log-rank P =3.18 × 10 −6 ). The median survival time for the AA genotype at rs4458204 was 11.5 years. SNPs in three other loci corresponding to regions around the transforming growth factor beta receptor II ( TGFBR2 ), interleukin 12B ( IL12B ) and interferon induced with helicase C domain 1 ( IFIH1 ) genes were found to be associated with breast cancer-specific death with FDR-adjusted P <0.10 ( Fig. 2 ). Figure 1: Quantile–quantile (QQ) plots of the observed P -values for association in the discovery stage. QQ plot of the observed −log10 P -values ( y axis) versus the ‘expected’ −log10 rank P -values ( x axis) for trend tests of association of 7,020 human immunology and inflammation SNPs, with the risk of dying from breast cancer for all ER-negative breast cancer patients (black/below) and ER-negative patients treated with adjuvant chemotherapy (blue/above) (genomic inflation factor, λ =1.16 and 1.14, respectively) in the discovery phase. The grey region indicates bootstrapped 95% confidence intervals. The diagonal red line indicates expected results under null hypothesis. The dotted lines indicate Bonferroni threshold for multiple-testing correction (2,184 independent tests with r 2 <0.2). Full size image Table 1 Summary of results for association of rs4458204_A with risk of dying from breast cancer. Full size table Figure 2: Manhattan plot for association in the discovery stage. Manhattan plot showing directly genotyped SNPs plotted according to chromosomal location ( x axis), with −log10 P -values ( y axis) derived from trend tests of association of 7,020 human immunology and inflammation SNPs with the risk of dying from breast cancer for all ER-negative patients (above) and ER-negative patients treated with chemotherapy (below) in the discovery phase. Blue and red lines indicate the Bonferroni threshold for multiple-testing correction for 2,184 ( r 2 <0.2) and genome-wide significance level (5 × 10 −8 ), respectively. SNPs with FDRs of <10% are additionally encircled and denoted in green. Chromosomal positions are based on NCBI build 36. Full size image Figure 3: Linkage disequilibrium plot of SNPs within a 100-kb window flanking rs4458204 in the discovery phase. The closest SNP flanking the left of rs4458204 is >9.5 Mb away. Chromosomal positions are based on NCBI build 36. P -values are derived from trend tests of association. 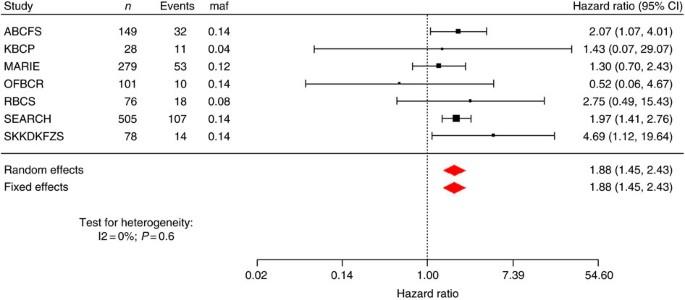Figure 4: Forest plot of a subset of studies in the discovery phase with at least ten events for rs4458204_A annotated to theCCL20gene. We found no evidence of heterogeneity in the per-allele HR across 14 studies (I2=0%,Pfor heterogeneity=0.84).P-value for both fixed and random effects meta-analyses on all 14 studies was 3.93 × 10−7, whereas on this reduced data set (studies with <10events excluded for clarity of presentation) it was 1.76 × 10−6, which passes the preset Bonferroni threshold of 2.29 × 10−5for 2,184 independent tests. The 95% confidence interval for each study is given by a horizontal line, and the point estimate is given by a square whose height is inversely proportional to the s.e. of the estimate. The summary odds ratio is drawn as a diamond with horizontal limits at the confidence limits and width inversely proportional to itss.e. Plotted using ‘snp.plotter’ package in R. Full size image Figure 4: Forest plot of a subset of studies in the discovery phase with at least ten events for rs4458204_A annotated to the CCL20 gene. We found no evidence of heterogeneity in the per-allele HR across 14 studies ( I 2 =0%, P for heterogeneity=0.84). P -value for both fixed and random effects meta-analyses on all 14 studies was 3.93 × 10 −7 , whereas on this reduced data set (studies with <10events excluded for clarity of presentation) it was 1.76 × 10 −6 , which passes the preset Bonferroni threshold of 2.29 × 10 −5 for 2,184 independent tests. The 95% confidence interval for each study is given by a horizontal line, and the point estimate is given by a square whose height is inversely proportional to the s.e. of the estimate. The summary odds ratio is drawn as a diamond with horizontal limits at the confidence limits and width inversely proportional to itss.e. 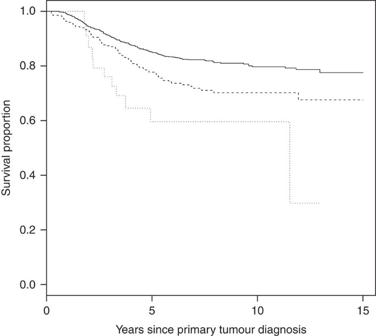Figure 5: Kaplan-Meier survival curves of breast cancer-specific survival in estrogen receptor-negative patients treated with chemotherapy for rs4458204 in the discovery phase. Analysis were adjusted only for time of blood draw and stratified by genotype. The p-value shown is based on the log-rank test. The number of events/n for each genotype are in parenthesis as follows rs4458204_GG (195/1415, single continuous line), rs4458204_AG (73/357, broken line) and rs4458204_AA (11/32, dotted line). The log rankP-value for this analysis was 3.18 x 10−6. Full size image Figure 5: Kaplan-Meier survival curves of breast cancer-specific survival in estrogen receptor-negative patients treated with chemotherapy for rs4458204 in the discovery phase. Analysis were adjusted only for time of blood draw and stratified by genotype. The p-value shown is based on the log-rank test. The number of events/n for each genotype are in parenthesis as follows rs4458204_GG (195/1415, single continuous line), rs4458204_AG (73/357, broken line) and rs4458204_AA (11/32, dotted line). The log rank P -value for this analysis was 3.18 x 10 −6 . Full size image From our replication study of rs4458204_A using multi-ethnic iCOGS Asian samples (522 ER-negative patients treated with chemotherapy, 53 events; see Supplementary Table 3 ), the per-allele HR after controlling for tumour characteristics and treatment was 1.97 (0.94–4.17); P for trend=0.07, Table 1 ). Together with multivariable-adjusted results from a second replication of the SNP using early-onset breast cancer patients POSH study, significant evidence of replication was observed (combined per-allele HR=1.52 (1.07–2.15), P for trend=0.02, Table 1 ). From a meta-analysis of both discovery and replication stages, the association of the SNP with risk of dying from breast cancer was found to be 1.81 (1.49–2.19; P for trend=1.90 × 10 −9 ) with no observed heterogeneity ( I 2 =1.4%, P for heterogeneity=0.36; Table 1 ). The cluster plots for the most significant SNP in our analysis, rs4458204 ( CCL20 ), and three other index SNPs of loci for which the associated test statistic passed FDR<0.1, namely rs1367610 ( TGFBR2 ), rs2569254 ( IL12B ) and rs13422767 ( IFIH1 ), were examined. All SNPs showed good discrimination of the three genotypes in cluster plots for the BCAC samples that passed quality control in the parent COGS study ( Fig. 6 ). 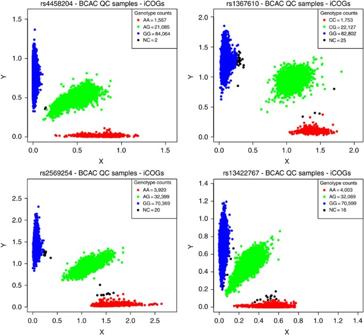Figure 6: Cluster plots of noteworthy SNPs. Cluster plots are shown for rs4458204 (CCL20), rs1367610 (TGFBR2), rs2569254 (IL12B) and rs13422767 (IFIH1) for the BCAC samples that passed quality control in the parent COGS study18. The SNP genotypes have been assigned based on cluster formation in scatter plots of normalized allele intensities X and Y. Each circle represents one individual’s genotype. Blue and red clouds indicate homozygote genotypes for the SNP (AA/aa), green heterozygote (Aa) and black undetermined. Three distinct, tight clusters exhibited by all four representative SNPs indicate good discrimination of the three genotypes. Figure 6: Cluster plots of noteworthy SNPs. Cluster plots are shown for rs4458204 ( CCL20 ), rs1367610 ( TGFBR2 ), rs2569254 ( IL12B ) and rs13422767 ( IFIH1 ) for the BCAC samples that passed quality control in the parent COGS study [18] . The SNP genotypes have been assigned based on cluster formation in scatter plots of normalized allele intensities X and Y. Each circle represents one individual’s genotype. Blue and red clouds indicate homozygote genotypes for the SNP (AA/aa), green heterozygote (Aa) and black undetermined. Three distinct, tight clusters exhibited by all four representative SNPs indicate good discrimination of the three genotypes. Full size image rs4458204 is located ~41.5 kb upstream of the chemokine (C–C motif) ligand 20 ( CCL20 ) gene. Chemokines are important mediators of immune response, and CCL20 has previously been shown to induce migration and proliferation of breast epithelial cells [28] . CCL20 has also been reported to be strongly chemotactic for lymphocytes and weakly attracts neutrophils [29] . However, rs4458204 was not found to be a significant ( P for trend>0.05) expression trait quantitative locus in any of the tissues (that is, adipose subcutaneous, artery tibial, blood, heart, lung, muscle skeletal, nerve tibial, skin and thyroid) reported on the publicly available Genotype-Tissue Expression Portal [30] . It is of note that the association of rs4458204_A with the survival of ER-negative breast cancer patients treated with chemotherapy increased and the strength of the association became stronger after adjustment for tumour characteristics and type of treatment (per-allele HR (95% confidence interval) from 1.64 (1.31–2.05) to 1.96 (1.55–2.47), P for trend from 1.27 × 10 −5 to 1.60 × 10 −8 ). This suggests that tumour characteristics and treatment covariates are likely to be confounders and thus it is desirable to include them in the fully adjusted model to obtain a more accurate effect size of the genetic factor. Moreover, it has also been shown that adjustment for prognostic factors will lead to a gain in power for statistical analyses. Genes in other regions indentified by the less stringent FDR threshold ( TGFBR2 , IL12B and IFIH1 ) have been implicated to play a role in breast cancer disease progression, suggesting that there are potentially more variants in immune response and inflammation genes that are associated with breast cancer prognosis. Although TGFBR2 is a breast cancer susceptibility locus [18] , none of the SNPs annotated to this gene was significantly associated with breast cancer risk ( P >0.05) in the parent COGS study. Although several GWAS have aimed to find genetic markers associated with breast cancer survival to date [22] , [31] , [32] , [33] , few credible variants have been robustly identified. The threefold greater breast cancer mortality for affected sisters is comparable in magnitude to the familial relative risk for breast cancer incidence, for which close to 100 independent susceptibility loci based on common variants (SNPs) have been identified, and these explain only a small proportion of familial aggregation of risk [18] . The failure to identify a similar number of survival-associated loci influencing survival may reflect the much lower statistical power for survival analyses to date, but may also reflect the substantial heterogeneity in tumour characteristics and treatment. As such, it has been suggested that sufficiently powered studies investigating specific cancer subtypes or treatment subgroups would need to be much larger to discover more regions in the genome associated with breast cancer prognosis [33] . In agreement, the association between rs4458204 and breast cancer survival for this study was found to be more pronounced (larger HR) for women with ER-negative disease treated with chemotherapy ( Table 1 ). However, as we did not study the association for women with ER-positive disease, the impact of this SNP on survival for those women remains unclear. One of the strengths of our study is that we have based our gene selection on commercially pre-designed panels of genes known to be differentially expressed in immunology and inflammation, which covers a comprehensive and validated list of relevant genes. The use of the iCOGS array in the BCAC consortium allowed us to investigate genetic variation across >500 immune response genes and provided an unprecedented large sample size with detailed clinical information to examine their associations with breast cancer survival. The results were also replicated by the POSH study, which is not part of the COGS consortium. However, SNPs related to immune response and inflammation were not specifically selected to be put on the iCOGS panel to give comprehensive coverage of these genes; only 557 of the 597 genes (~93%) were represented. The proportion of total phenotypic variance (Nagelkerke pseudo R -squared) explained by this SNP alone was also small, at ~1.3%, suggesting that many more variants will need to be discovered for such genetic data to be useful in a clinical setting. Our findings suggest that host factors affecting the ability to respond to systemic treatment or to mount an effective immunologic response contribute to the heritability of prognosis. Such survival-associated variants can represent ideal targets for tailored therapeutics and may also enhance our current prognostic prediction capabilities. How to cite this article: Li, J. et al . 2q36.3 is associated with prognosis for oestrogen receptor-negative breast cancer patients treated with chemotherapy. Nat. Commun. 5:4051 doi: 10.1038/ncomms5051 (2014).